Provable quantum advantage in randomness processing Quantum advantage is notoriously hard to find and even harder to prove. For example the class of functions computable with classical physics exactly coincides with the class computable quantum mechanically. It is strongly believed, but not proven, that quantum computing provides exponential speed-up for a range of problems, such as factoring. Here we address a computational scenario of randomness processing in which quantum theory provably yields, not only resource reduction over classical stochastic physics, but a strictly larger class of problems which can be solved. Beyond new foundational insights into the nature and malleability of randomness, and the distinction between quantum and classical information, these results also offer the potential of developing classically intractable simulations with currently accessible quantum technologies. Suppose you are handed a classical coin with some unknown bias, is there a method by which one can simulate a perfectly fair coin-flip? A popular method (often attributed to von-Neumann [2] ) is as follows: flip the coin twice, if the two outcomes are different then output the coin with its value on the second flip, otherwise start over. Provided that the unknown probability of heads, p is not 0 or 1, it is clear that this method yields, with probability one, an unbiased output after a random number of coin-flips. Contrast this with the case where one is asked to output a new coin that has probability of heads p 2 . In this case exactly two flips suffice for any p ∈ [0, 1]: we flip the biased coin twice and if both flips are heads then we output the new coin showing heads, otherwise we output it showing tails. These two examples tell us that the output bias functions f ( p ):=1/2 and f ( p ):= p 2 can both be ‘constructed’ by flipping a coin with some unknown bias p . More generally, we say that a function f is constructible if there is an algorithm that yields an output with bias f ( p ), almost surely after a finite number of coin-flips. Slightly more precisely: for all p the procedure to construct f ( p ) must define disjoint sets S 1 and S 2 whose elements are finite strings, such that with probability 1 the sequence of flips produced has exactly one of these strings as an initial segment. For any sequence of flips the output is heads if the initial segment is in S 1 and tails if it is in S 2 , and thus an output is produced almost surely in finite time. In the mathematics literature the words observable and simulable are often used, however these already have unrelated and so potentially confusing technical meaning within quantum theory. The topic of which functions are constructible, how easily they can be constructed, and their applications goes by the name ‘Bernoulli Factory’ [2] , [3] , [4] , [5] . Crucially, in 1995 a theorem of Keane and O'Brien [2] determined the exact set of functions constructible from a classical coin of unknown bias p . Loosely speaking, it was found that a function f ( p ):( S [0, 1])→[0, 1] is constructible if and only if (a) it is continuous, (b) it does not touch 0 or 1 within its domain and (c) it does not approach zero or one exponentially quickly at any edge of its domain (see the Supplementary Methods for a precise statement). While this allows such surprising functions as , it also rules out important ones such as as the ‘probability amplification’ function f ( p )=2 p , which is central to certain stochastic simulation protocols. Moreover, it says nothing about the resources required to actually construct the functions—often an infeasibly large number of coin-flips are required. The scenario described for the Bernoulli factory bears similarities to a Turing Machine, however it is worth emphasizing that there are differences between them. While both possess a target function to be ‘computed’, the Bernoulli factory, with its unbounded, probabilistic, identically independently distributed input, is in a sense a simpler, arguably more tractable, model. This makes the Bernoulli Factory an ideal candidate with which to establish quantum-mechanical results that are provably beyond the reach of classical physics. There are two central results presented in this work. Firstly, the Quantum Bernoulli Factory (QBF) allows the construction of a strictly larger class of functions than allowed in stochastic classical physics. Secondly, the QBF provides dramatic improvements in terms of resource requirements over a range of classically constructible functions. 2 p protocol The classical Bernoulli Factory (CBF) can be easily described within a quantum-mechanical setting via (arbitrarily many) copies of a qubit prepared in the mixed qubit state for unknown p ∈ S [0, 1]. Here the computational basis of the two-dimensional qubit Hilbert space , denotes a fiducial projective measurement that extracts classical data. In contrast, a quantum-mechanical extension of the classical coin states has coherences in this basis. Our goal is to contrast the fundamental processing of such classical randomness with the quantum randomness attainable in a QBF. It should be emphasized, however, that our desired output is still classical. We refer to the quantum-mechanical extension of the coin state as a quoin, and accordingly it is described by the coherent state For this we find measurement in the computational basis returns the probability distribution ( p , 1− p ), and so by restricting to stochastic mixing in this basis, together with algorithmic processing, we see that the CBF setting is recovered as a special case from the quantum-mechanical one. In particular we see that the stochastic mixing available in the classical factory is a special case of the unitary operations available in the quantum setting. One could consider convex combinations of unitaries, however this turns out to be equivalent, since it is always possible to simulate this stochasticity via unitary generation of randomness on a subset of quoins or ancillae qubits. We now demonstrate that the full set of quantum-mechanical operations allows a strictly larger class of functions than allowed classically. We focus on the primary example studied in the CBF literature, the probability amplification function f ( p )=2 p . This function is impossible to construct classically, since it attains the value f ( p )=1 for p =1/2, and so traditional work-arounds involve ‘chopping’ the function as it approaches p =1/2, and forming a truncated function, f ( p )=min(2 p , 1−ɛ) for some fixed 0<ɛ<1. This approximate function then does satisfy the conditions of the Keane O'Brien theorem, however the amount of coins needed to produce such a function scale very poorly with ɛ (see refs 6 , 7 for examples). By contrast we will now show that within a QBF it is possible to efficiently construct the classically impossible probability amplification function f :[0, 1]→[0, 1] defined by: as shown in Fig. 1 . 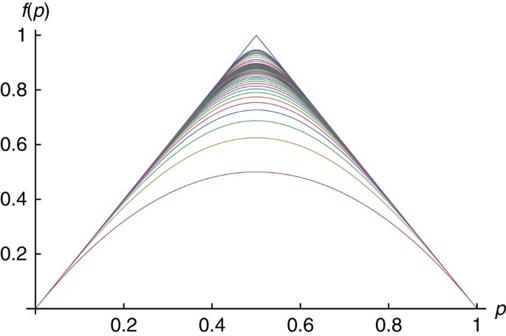Figure 1: The probability amplification function. This figure shows the amplification functionf:[0, 1]→[0, 1], and the first 35 functions in the convex decomposition (3). This function is impossible to construct classically, but can be achieved quantum mechanically via two-qubit measurements in the entangled Bell-basis, together with classical processing. Figure 1: The probability amplification function. This figure shows the amplification function f :[0, 1]→[0, 1], and the first 35 functions in the convex decomposition (3). This function is impossible to construct classically, but can be achieved quantum mechanically via two-qubit measurements in the entangled Bell-basis, together with classical processing. Full size image Our method is as follows. The target function admits an alternative representation of , which in turn possesses an expansion of the form where q k is a probability distribution independent of p . Since within the CBF or QBF we can generate any constant distribution, we first construct an integer output k with probability and then conditioned on this output construct the function g k ( p )=(4 p (1− p )) k . The latter set of functions { g k } are classically inaccessible for all k >0. We also note that and so our task reduces to constructing the k =1 case. This is easily achieved by considering a Bell-basis measurement on two quoins . The probability that we obtain or is 1/2, however the probability of obtaining the outcome , conditioned on obtaining or is exactly 4 p (1− p )≡ g 1 ( p ). Putting everything together, to construct a f ( p ) coin we output an index k with probability q k and then construct k g 1 ( p )-coins using quoins. If k outcomes of heads in a row are obtained from the g 1 ( p )-coins then heads is output, otherwise tails is output. This provides an exact construction of the function f , as claimed. We can provide a clearer account of this construction by adapting a method in [8] , where we can represent the above method as a random walk on a ladder as depicted in Fig. 2 . One begins at the point marked Start and flips a g 1 ( p )-coin to decide where to move next. Once on the ladder at any vertex we step up the ladder with probability g 1 ( p )/2, or down the ladder with the same probability; otherwise we move across. If we reach the bottom left corner we output heads, while if we reach the bottom right corner we output tails; this means that if the very first flip is tails we output tails immediately. 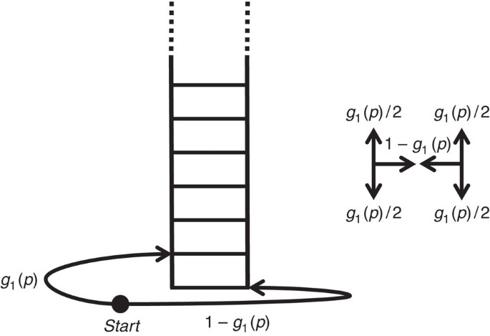Figure 2: The random walk used in the 2pprocedure. The quantum probability amplification construction can be represented via a random walk on a semi-infinite ladder with transitions given by Bell-measurement outcomes on two qubits. The bell procedure gives a result of heads with probabilityg(p). Initially one flip is used to determine the starting point. After the first flip a result of heads causes a move upwards or downwards with equal probability; a result of tails causes a move to the other side of the ladder. If the bottom left corner is ever reached, we output heads, if the bottom right is reached we output tails. The probability of outputting heads overall is. The probability of outputting heads can be shown to be Figure 2: The random walk used in the 2 p procedure. The quantum probability amplification construction can be represented via a random walk on a semi-infinite ladder with transitions given by Bell-measurement outcomes on two qubits. The bell procedure gives a result of heads with probability g ( p ). Initially one flip is used to determine the starting point. After the first flip a result of heads causes a move upwards or downwards with equal probability; a result of tails causes a move to the other side of the ladder. If the bottom left corner is ever reached, we output heads, if the bottom right is reached we output tails. The probability of outputting heads overall is . Full size image The construction that we have provided uses two-qubit measurements in an entangled basis, and so one might think that entanglement is required for any quantum advantage; surprisingly this is not the case—the following theorems determine the exact class of functions f :[0, 1]→[0, 1] that are constructible within a QBF using only single-qubit operations, and are the main results of this work. In fact the only type of operations required for our proofs are the unitaries which construct a coin that gives output one with probability Classes of constructible functions Theorem 1 : a function f :[0, 1]→[0, 1] is constructible with quoins and a finite set of single-qubit operations if and only if the following conditions hold: 1 is continuous. 2 Both Z ={ z i : f ( z i )=0} and W ={ w i : f ( w i )=1} are finite sets. 3 z ∈ Z there exists constants c , δ >0 and and integer k <∞ such that 4 w ∈ W there exist constants c , δ>0 and an integer k <∞ such that The proof of Theorem 1 is too long to include here and is provided in the Supplementary Methods . The main idea is similar to the construction of the probability amplification function, and involves arriving at a convex decomposition in terms of functions that are explicitly constructible using quantum operations on quoins. The proof is constructive although far from optimal. It is clear that the conditions of the theorem are a natural generalization of the classical case, except now the function is allowed to go (polynomially quickly) to 0 and 1 at a finite number points over the interval [0, 1]. Moreover, this implies that the scaling of resources within the interior no longer behaves as in the classical case, where large number of coins is required if the function approaches 0 or 1 at, for example, p =1/2 for f ( p ). One straightforward generalization is that we do not require the target function be defined at all points inside the interval [0, 1], and can allow more extreme behaviours (such as rapidly increasing oscillations or apparent discontinuities) in the functions that we construct, see Fig. 3 . To this end we have the following theorem. 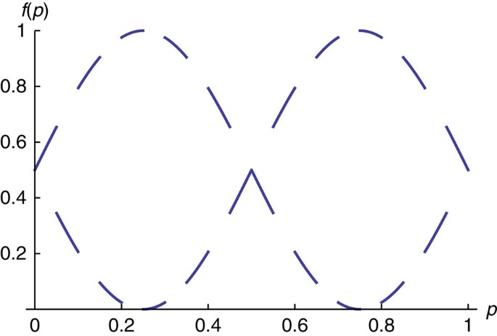Figure 3: One example of a constructible function which appears discontinuous. One example of the unusual functions one could construct using Theorem 2, the actual discontinuities are excluded. Effectively we gain access to piecewise continuous functions but with their discontinuous points excluded, leaving a function which is continuous on its domain. Figure 3: One example of a constructible function which appears discontinuous. One example of the unusual functions one could construct using Theorem 2, the actual discontinuities are excluded. Effectively we gain access to piecewise continuous functions but with their discontinuous points excluded, leaving a function which is continuous on its domain. Full size image Theorem 2 : A function f :(0, a 1 ) ∪ ( a 1 , a 2 ) ∪ ... ∪ ( a n , 1)→[0, 1] is constructible with quoins and a finite set of single-qubit unitaries if f is continuous on its domain and there exists a finite list { a 1 , a 2 , ... a n ′ }, which contains { a 1 , a 2 , ... a n }, and integer k such that for all p ∈ (0, 1), where The proof of Theorem 2 follows a slightly different construction to Theorem 1, and is also provided in the Supplementary Methods . As before, the proof is constructive but far from optimal. The above two theorems both relate to single-qubit operations and provide a broad class of constructible functions, however multi-qubit unitaries do not extend the set of quantumly constructible functions, but do provide additional speed-ups, as is illustrated by the example of the function g 1 ( p ) constructed from Bell measurements. In addition to extending the class of constructible functions, the quantum-mechanical Bernoulli Factory provides dramatic speed-ups for certain functions that are classically accessible. For example, consider the function with 0< α <1, which is easily constructed via a convex combination of h a (which requires just a single quoin) and the function 0. Since the function h a is inaccessible classically, the construction of the function f α necessarily requires a rapidly increasing number of classical coins as α tends to 1, in stark contrast to the quantum-mechanical case which requires only a single quoin for all values of α . This leads us to argue that unlike many black-box scenarios, such as the Deutsch–Jozsa algorithm [9] , our advantage survives the addition of errors. Since the classical coin requirements scale exponentially [6] with the cutoff ɛ at the top of the f ( p ) function, it would be impossible in the presence of any realistic errors for the classical factory to catch up for small values of ɛ . Another obvious question is when do we find ourselves in a position where we have a superposition of a probability distribution but the actual distribution is unknown to us. Recent work on boson sampling [10] provides an example of just that. The circuit is extremely hard to classically simulate and quantum mechanically we can only sample from the distribution, not efficiently learn it. If one wanted to perform some transformation on the distribution the quantum Bernoulli factory would certainly be applicable. This is just one of several avenues [11] , [12] , [13] , [14] , [15] , [16] , [17] , [18] where the quantum Bernoulli factory might offer insight. The distinguishing features of quantum and classical information are subtle, and often well-hidden. Paradigmatic examples have already appeared in single-party cryptography [19] , two-party cryptography and communication complexity [20] . Of arguably broader significance is to determine the computational abilities allowed by quantum physics. Quantum computing does not allow new functions to be constructed and the speed-ups, whilst strongly supported by evidence remain unproven. The work presented here provides a computational scenario in which quantum mechanics has strict superiority over classical physics, and by virtue of requiring only single-qubit manipulations appears vastly easier to attain experimentally. Understanding models like this one will lead to a better understanding of quantum computing. How to cite this article: Dale, H. et al . Provable Quantum Advantage in Randomness Processing. Nat. Commun. 6:8203 doi: 10.1038/ncomms9203 (2015).